Magnetic properties of uncultivated magnetotactic bacteria and their contribution to a stratified estuary iron cycle Of the two nanocrystal (magnetosome) compositions biosynthesized by magnetotactic bacteria (MTB), the magnetic properties of magnetite magnetosomes have been extensively studied using widely available cultures, while those of greigite magnetosomes remain poorly known. Here we have collected uncultivated magnetite- and greigite-producing MTB to determine their magnetic coercivity distribution and ferromagnetic resonance (FMR) spectra and to assess the MTB-associated iron flux. We find that compared with magnetite-producing MTB cultures, FMR spectra of uncultivated MTB are characterized by a wider empirical parameter range, thus complicating the use of FMR for fossilized magnetosome (magnetofossil) detection. Furthermore, in stark contrast to putative Neogene greigite magnetofossil records, the coercivity distributions for greigite-producing MTB are fundamentally left-skewed with a lower median. Lastly, a comparison between the MTB-associated iron flux in the investigated estuary and the pyritic-Fe flux in the Black Sea suggests MTB play an important, but heretofore overlooked role in euxinic marine system iron cycle. Since the discovery of magnetotactic bacteria (MTB) 50 years ago [1] , [2] , these microorganisms have continued to captivate the attention of geoscientists with their remarkable diversity, metabolic flexibility, magnetism and ubiquity. The observation that chemically stratified euxinic basins host thriving populations of MTB [3] , [4] , [5] , [6] , [7] has led to the proposition that magnetosomes are an important component of the euxinic system iron cycle and can serve as biomarkers of past ocean redox shifts [8] , [9] . The suggestion that MTB play an important role in the iron cycle stems from the fact that iron must be sequestered from the surrounding environment in order for them to biosynthesize their iron-rich organelle [6] , [10] . Some of the magnetosome-bound iron can be released back into the environment via ingestion and subsequent digestion of MTB by protozoan [10] , [11] or by dissolution with or without assistance by the iron-chelating siderophores MTB produce themselves [8] , [10] , [12] , [13] , while the rest can be incorporated as intact magnetosomes into the sedimentary matrix. As for their relevance as a redox proxy, there are at least two possible scenarios. First, as MTB population size tends to scale with the width of the chemocline [14] , sedimentary magnetofossil concentration can reflect changes in chemocline width in response to deoxygenation and recovery. Second, as greigite-producing MTB require sulphur for magnetosome biosynthesis [8] , their occurrences are probably correlated with the many episodic euxinia experienced by the Earth’s ocean in the geological past [15] . As such, the presence of greigite (Fe 3 S 4 ) magnetofossils in geological records has been suggested as an indicator of euxinia [8] , [9] , [16] , [17] . Ascertaining the role MTB play in stratified euxinic systems’ iron cycle requires knowledge of the amount and rate of magnetosome-bound iron that can be exported out of the oxic–anoxic interface (OAI), where high abundance of live MTB are found in such chemically stratified environments. The former has been estimated for one meromictic coastal salt pond [6] , [7] , but a quantitative assessment of the latter has not been forthcoming. Furthermore, for magnetofossils to serve as a marker of paleo-redox conditions, there must be accurate ways of detecting them in the geological records and an understanding of how diagenesis affects their concentration in sediments. Magnetofossil detection methods employing magnetic property measurements in use today are largely based on characterizations of MTB isolated in pure culture known to produce linear chains of magnetite (Fe 3 O 4 ) magnetosomes [18] , [19] , [20] , [21] , [22] , [23] , [24] , [25] , [26] . Mechanistically, these methods are founded on the low-temperature crystallographic transition specific to single-magnetic domain magnetite [18] , pronounced uniaxial magnetic anisotropy that arises from the magnetosome chain architecture [20] , [21] , [22] , [23] , [24] , [25] , [26] , [27] , [28] and the uniformity in magnetosome size [19] . Characterized MTB cultures, however, are not representative of the diverse and naturally occurring magnetosome geometry, crystallography and mineralogy that can ultimately be preserved in the geological records. For example, the only greigite-producing MTB recently cultivated in the laboratory, strain BW-1, biosynthesizes either single or double chains of magnetite and/or greigite, depending on hydrogen sulphide concentration and/or redox potential in the growth medium [29] . BW-1 represents just one of the two known greigite-producing MTB morphotypes and has never been characterized by any of the magnetofossil detection method in use today. There is also a lack of magnetic characterization on similar but uncultivated greigite-producing MTB large rods, as well as the other known greigite-producing MTB, multicellular magnetotactic prokaryote, all of which commonly produce disaggregated magnetosome clusters and bundles [3] , [4] , [30] , [31] , [32] , [33] , [34] . Non-chain magnetosome geometry is not restricted to greigite-producing MTB, as there have been numerous reports of uncultivated magnetite-producing MTB that do not form simple single chains [35] and whose magnetic properties remain largely unknown. As such, there are major open questions concerning the applicability of existing methods for detecting greigite magnetofossils and magnetofossils not arranged in simple single chains [36] . Here we have collected uncultivated live MTB that have not yet been subjected to diagenesis from the stratified water column of Upper Pond, Pettaquamscutt River Estuary, Rhode Island, USA. We report ferromagnetic resonance (FMR) and coercivity distribution characterizations on collections of uncultivated MTB that produce magnetite, co-produce greigite and magnetite, and only greigite. We show that uncultivated MTB are characterized by a wider range of FMR empirical spectral parameters compared with the five cultured magnetite-producing MTB strains that have been characterized to date [20] , [21] , [22] , [25] , [26] , [36] , [37] . We also show that compared with putative Neogene greigite magnetofossil-bearing sedimentary rocks [16] , [38] , the coercivity distributions of uncultivated MTB that produce magnetite, magnetite and greigite, or greigite only, are fundamentally left-skewed with a lower median. We consider the implications these new FMR and coercivity distribution results have on magnetofossil detection and quantification. We conclude by determining the MTB population turnover rate in Upper Pond and discuss the role MTB play in the euxinic system iron cycle. Layered MTB population in the water column We collected uncultivated MTB as a function of water depth, d , from the Upper Pond, Pettaquamscutt River Estuary ( Fig. 1 ). The Upper Pond (maximum depth 13.5 m, surface area 0.29 km 2 ) is one of two brackish basins, separated from one another by shallow sills, located in North Kingstown, Rhode Island, USA [39] . Except for the complete water column overturn that occurs every 5 to 10 years [39] , the water column stratification in Upper Pond is maintained year-round mainly by the salinity contrast between its two water sources: the Gilbert Stuart Stream and the Rhode Island Sound [39] . The bottom water of both basins in the Pettaquamscutt River Estuary is depleted in dissolved oxygen (DO), due to aerobic heterotrophic respiration and the limited atmospheric oxygen downward diffusion, and enriched in hydrogen sulphide (H 2 S) generated by anaerobic microbial sulphate reduction [4] , [39] , [40] . In two previous studies carried out in the Lower Pond [3] , [4] , the other brackish basin in the Pettaquamscutt River Estuary located ~1 km south of our sampling site, the highest number of live MTB were found around the OAI. Among at least seven MTB morphotypes observed in the Lower Pond [3] , [4] , a vibrio (MV-2) and a coccus (MC-1) MTB strain were isolated in axenic culture, both of which are producers of single-chain magnetite magnetosomes [41] , [42] , [43] . The other observed MTB morphotypes have not been cultivated, including one that simultaneously produces magnetite and greigite magnetosomes [3] , [4] . The MTB population in the Lower Pond water column has a layered structure: magnetite producers are found in the microaerobic to anaerobic depth, greigite producers are found in the anaerobic and sulphidic depth, and the magnetite and greigite co-producers are found below the magnetite producers but above the greigite producers [4] . 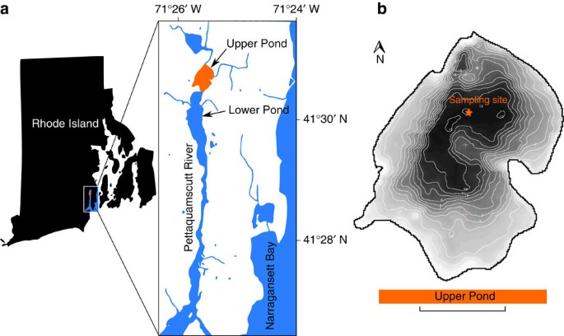Figure 1: Sampling site. (a) The location of Upper Pond in the Pettaquamscutt River Estuary, RI, USA. (b) Zoomed in bathymetry map of the Upper Pond. Scale bar, 1/4 km. Figure 1: Sampling site. ( a ) The location of Upper Pond in the Pettaquamscutt River Estuary, RI, USA. ( b ) Zoomed in bathymetry map of the Upper Pond. Scale bar, 1/4 km. Full size image DO and Eh measurements (Methods) show that on the day of our sampling the water column of Upper Pond was stratified with a well-developed OAI at d =5.2 m and support the presence of H 2 S below d =5.0 m ( Fig. 2a ). The sulphide concentration in Upper Pond has been measured directly in the past [39] , [40] . In the interval d =3.9–7.0 m, we observe abundant live MTB, as well as some magnetically responsive protists, directly by the hanging-drop assay ( Fig. 2b–d ; Methods). The assay shows a decrease in the MTB diversity and a change in MTB morphotype distribution with increasing water depth in agreement with an established MTB population structural model for euxinic basins [8] ; whereas fast-swimming cocci, barbell-shaped cells, small rods and vibroids are common in shallower microaerobic to anaerobic depths, slow-moving large rods dominate in deeper anaerobic and sulphidic depths ( Fig. 2b ). According to this MTB population structural model, magnetite producers inhabit the microaerobic to anaerobic zone, whereas greigite producers dwell in the sulphidic hypolimnion, which is compatible with the microscopy findings of Bazylinski et al. [4] from the Lower Pond. This distribution of MTB is thought to be governed by the thermodynamic stability of magnetite versus greigite with respect to the DO and H 2 S gradient [8] . 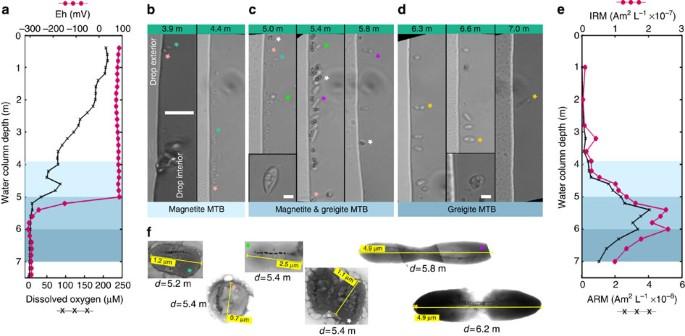Figure 2: Upper Pond water column profiles and microscopy observations. (a) Water column dissolved oxygen andEhmeasured on 15 September 2012. (b–d) Light microscopy hanging-drop live MTB assay images for selected water depths betweend=3.9–7.0 m where live MTB were observed. The 10-μm scale bar in (b) applies to all panels except for the lower magnification (50-μm scale bar) images of magnetic responsive protists shown in the insets of (c) and (d). All images were captured on the hanging-drop edge corresponding to North-seeking MTB. (e) Ferrimagnetic particle concentration-dependent parameters: IRM (200mT) and ARM (AFmax=200 mT, DC=0.1 mT). (f) TEM images of selected MTB cells. MTBs fromd=5.8 m andd=6.2 m are analysed for their magnetosome composition (seeFig. 3). The coloured stars mark probable MTB morphotype connection between the TEM images and the light-microscopy hanging-drop assay. Light, medium, dark shades of blue demarcate water column zones inhabited by magnetite MTB, mixed magnetite and greigite MTB and greigite MTB, respectively (see text). Figure 2: Upper Pond water column profiles and microscopy observations. ( a ) Water column dissolved oxygen and Eh measured on 15 September 2012. ( b – d ) Light microscopy hanging-drop live MTB assay images for selected water depths between d =3.9–7.0 m where live MTB were observed. The 10-μm scale bar in ( b ) applies to all panels except for the lower magnification (50-μm scale bar) images of magnetic responsive protists shown in the insets of ( c ) and ( d ). All images were captured on the hanging-drop edge corresponding to North-seeking MTB. ( e ) Ferrimagnetic particle concentration-dependent parameters: IRM (200mT) and ARM (AF max =200 mT, DC=0.1 mT). ( f ) TEM images of selected MTB cells. MTBs from d =5.8 m and d =6.2 m are analysed for their magnetosome composition (see Fig. 3 ). The coloured stars mark probable MTB morphotype connection between the TEM images and the light-microscopy hanging-drop assay. Light, medium, dark shades of blue demarcate water column zones inhabited by magnetite MTB, mixed magnetite and greigite MTB and greigite MTB, respectively (see text). Full size image Measurements of ferrimagnetic particle concentration-dependent parameters from filters containing water column particulates >0.22 μm present a broad peak bracketing the interval d =3.9–7.0 m ( Fig. 2e ; Supplementary Figs 12 and 18 ). Together with the negligible magnetic background from d =0–3.9 m ( Fig. 2e , and Supplementary Figs 12 and 18 ), where no live MTB were present as determined by the hanging-drop assay, we deduce that MTB are the principal carriers of the magnetic signal around the OAI. Using our hanging-drop assay results, the established MTB population structural model for euxinic basin described above [8] and the findings of Bazylinski et al. [4] from the nearby Lower Pond, we divide the Upper Pond water column into three broad MTB zones: (1) d =3.9–5.0 m, containing diverse morphotypes of magnetite-producing MTB; (2) d =5.0–6.0 m, containing MTB producing both magnetite and greigite; and (3) d >6.0 m, containing greigite-producing MTB. We validated our demarcation by performing analytical microscopy on MTB from d =5.8 m and d =6.2 m ( Fig. 3 ; Methods) and found excellent agreement. A bimodal distribution of Fe/S atomic ratios from energy dispersive X-ray (EDS) characterizes magnetosomes (number of analysed magnetosomes, n =38) in MTB from d =5.8 m, whereas Fe/S atomic ratios for those in MTB from d =6.2 m ( n =33) are uniformly low ( Fig. 3c ). The high and low Fe/S atomic ratio particles are indicative of magnetite and greigite, respectively. The majority of magnetosomes with low Fe/S atomic ratio in the bacterium from d =5.8 m and all of the magnetosomes in the bacterium from d =6.2 m are approximately square to rectangular in shape (in two-dimensional projection) and have non-uniform contrast ( Supplementary Fig. 1 ). The greigite magnetosomes identified in the study of Bazylinski et al. [4] from Lower Pond were associated with rectangular morphology. Non-uniform contrast is a common feature of greigite magnetosomes [30] , [31] , [32] , [33] . These features are thought to reflect either irregular particle surfaces or structural defects, with the latter hypothesized to have resulted from the transformation of machinawite or cubic FeS to greigite [30] . 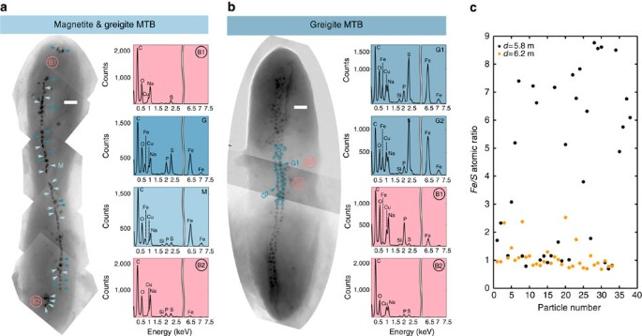Figure 3: Composition analyses on MTB magnetosomes and background membrane. (a)d=5.8 m and (b)d=6.2 m analysed with EDS. The particles in the magnetosome chain in the MTB fromd=5.8 m show an approximately binary distribution of atomic Fe/S ratio. We have interpreted particles with Fe/S>3 as magnetite magnetosomes (marked by light blue arrows next to the particles) and Fe/S<3 as greigite magnetosomes (marked by dark blue arrows next to the particles). In contrast, all of the particles analysed (blue ellipses) in MTB fromd=6.2 m have Fe/S<3 (c), which are probably greigite magnetosomes. EDS spectra are shown for selected representative particles/membrane as marked: G and M for greigite and magnetite magnetosomes in (a), respectively, and G1 and G2 both for greigite magnetosomes in (b). No EDS peaks were identified for 3<kV<6. B1 and B2 represent background cell membrane EDS signals. Figure 3: Composition analyses on MTB magnetosomes and background membrane. ( a ) d =5.8 m and ( b ) d =6.2 m analysed with EDS. The particles in the magnetosome chain in the MTB from d =5.8 m show an approximately binary distribution of atomic Fe/S ratio. We have interpreted particles with Fe/S>3 as magnetite magnetosomes (marked by light blue arrows next to the particles) and Fe/S<3 as greigite magnetosomes (marked by dark blue arrows next to the particles). In contrast, all of the particles analysed (blue ellipses) in MTB from d =6.2 m have Fe/S<3 ( c ), which are probably greigite magnetosomes. EDS spectra are shown for selected representative particles/membrane as marked: G and M for greigite and magnetite magnetosomes in ( a ), respectively, and G1 and G2 both for greigite magnetosomes in ( b ). No EDS peaks were identified for 3<kV<6. B1 and B2 represent background cell membrane EDS signals. Full size image Ferromagnetic resonance FMR spectroscopy is a non-destructive magnetofossil detection method that is sensitive to the net magnetic anisotropy resulting from factors such as particle size, shape, arrangement, composition and magnetostatic interactions. Its utility in magnetofossil detection is based on the observation that FMR spectra of intact magnetite single-chains from cultured MTB exhibit a number of distinguishing properties: multiple low-field absorption peaks in the derivative spectra and extracted empirical parameters from the integrated spectra that fall within a small range of values [20] , [21] , [22] , [24] , [25] , [37] demarcated by the dashed lines in Fig. 4a,b : effective g-factor g eff <2.12, asymmetry ratio A <1 and α <0.25. When the chains are randomly oriented and far apart, the low-field absorption peaks are related to resonance conditions satisfied by chains oriented parallel and perpendicular to the external field due to the positive uniaxial anisotropy [21] , [28] . The position of these peaks depends on the length of the chain: the longer the chains, the further apart the peaks become [20] , [44] . Both the g eff ≤2.12 (intrinsic g-factor for magnetite) and the low-field extended absorption, reflected in A <1, are also the result of the chain architecture [21] , [28] . The empirical parameter α combines measures of spectral asymmetry with the width of the absorption spectrum to estimate specimen heterogeneity. Intact magnetite single-chain magnetosomes from MTB cultures have α <0.25 (refs 21 , 22 , 24 ). 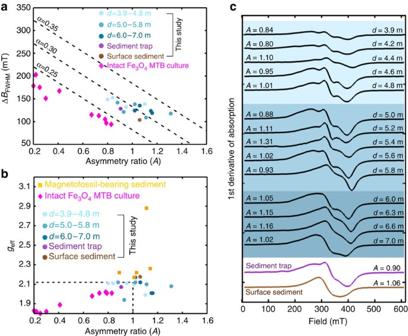Figure 4: FMR spectra and derived empirical parameters. (a,b) FMR empirical parameters from this study, cultured magnetite MTB20,21,22,24,25,37and magnetofossil-bearing sediments20,21. Intact magnetite MTB cultures are defined by the following parameters range:geff<2.12, asymmetry ratioA<1 andα<0.25. The parameters from this study fall within the range 0.80<A<1.31, 1.94<geff<2.17, 0.28<α<0.34. (c) FMR absorption derivative spectra (with compressed ordinate scaling) from water column filters, sediment trap and surface sediment samples. Figure 4: FMR spectra and derived empirical parameters. ( a , b ) FMR empirical parameters from this study, cultured magnetite MTB [20] , [21] , [22] , [24] , [25] , [37] and magnetofossil-bearing sediments [20] , [21] . Intact magnetite MTB cultures are defined by the following parameters range: g eff <2.12, asymmetry ratio A <1 and α <0.25. The parameters from this study fall within the range 0.80< A <1.31, 1.94< g eff <2.17, 0.28< α <0.34. ( c ) FMR absorption derivative spectra (with compressed ordinate scaling) from water column filters, sediment trap and surface sediment samples. Full size image We characterize filters containing collections of uncultivated MTB from the Upper Pond water column by room-temperature FMR spectra using a Bruker EPR spectrometer operating at X-band (Methods). MTB in the Upper Pond water column as a whole are characterized by a wider range of empirical FMR parameters (0.80< A <1.31, 1.94< g eff <2.17, 0.28< α <0.34) than intact cultured magnetite MTB ( Fig. 4a,b and Supplementary Table 6 ). 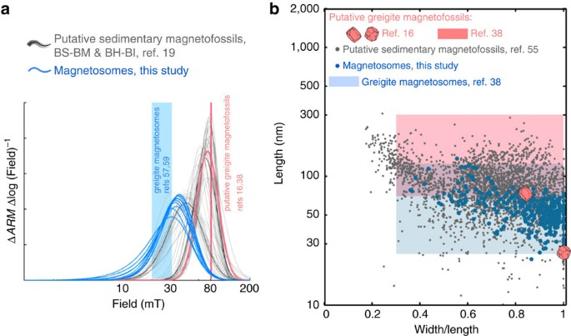Figure 6: Coercivity distribution and magnetosome size and shape. (a) Blue curves: ARM coercivity distribution of the water column samples from this study. Grey curves: hypothesized sedimentary magnetofossil coercivity distribution components BS-BM and BH-BI19. Black curves: averaged BS-BM and BH-BI. Thick light blue band: average coercivity determined from pulse-field experiments on individual greigite MTB from refs57,59. Thin magenta band: approximate median coercivity from a Miocene marl in ref.38containing greigite with similar crystal size distribution as MMP (‘many-celled magnetotactic prokaryote’), a greigite-producing MTB. Magenta curve: coercivity distribution determined from IRM acquisition curve unmixing from Pliocene sediment containing putative greigite magnetofossils16. (b) Aspect ratio (width/length) versus length for 377 magnetosomes imaged from 21 MTB in this study (blue dots). The grey dots (n~3000) are measured length and aspect ratio from putative magnetofossils extracted from marine and lacustrine sediments55. Blue and magenta boxes mark the length and aspect ratio ranges for MMP magnetosomes and greigite from the Miocene marl sample mentioned above, respectively, from ref.38. Magenta symbols denote magnetofossil shapes for the claimed oldest greigite magnetofossils from ref.16. In zone 1 where magnetite-producing MTB dominate, we observed multiple low-field absorption peaks ( Fig. 4c ). The small cocci and barbell-shaped MTB cells in this zone produce short magnetosome chains ( Fig. 2b,f ), which explains the close peak positions. However, Fig. 4c shows that such peaks are absent from samples in zone 3, where greigite-producing large rods dwell in the stratified water column. Direct transmission electron microscopy (TEM) observation from a greigite-producing MTB from d =6.2 m shows that the magnetosomes are close to one another and not organized in a single chain within the cell ( Fig. 3b and Supplementary Fig. 1b ). As such, we attribute the lack of multiple low-field peaks for spectra in zone 3 to magnetostatic interactions between magnetosomes. This interpretation is consistent with the reduced remanence ratios ( χ ARM /IRM) of 1.3–1.6 m mA −1 ( Supplementary Fig. 6 ) and non-negligible first-order-reversal curve (FORC) contribution in the H u >0 space ( Fig. 5 and Supplementary Fig. 14 ) that characterize zone 3 filters. MTB with isolated single chains typically have χ ARM /IRM=2.5–3.5 m mA −1 (refs 18 , 21 ) and negligible FORC contribution in the H u >0 space [26] . 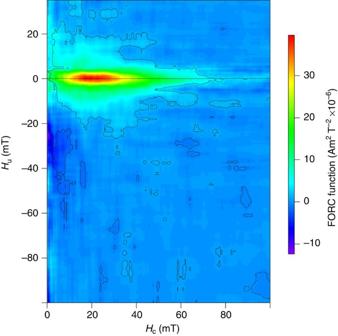Magnetostatic interaction is known to produce FMR spectral broadening [22] , [44] , [45] , reduce the χ ARM /IRM ratio [22] , [46] and increase FORC contribution in the H u >0 space [47] . Figure 5: First-order reversal curves diagram from greigite MTB. The measurement was made on a stack of filters containing >0.22 μm particulate filtered from 330 ml of water fromd=6.6 m. Five identical sets of raw data were averaged and processed with a variable smoothing grid:Sc=15,Su,0=10,Su,1=15,λH=0.1. The dotted contours denote FORC distributions that are significant at the 0.05 level. Figure 5: First-order reversal curves diagram from greigite MTB. The measurement was made on a stack of filters containing >0.22 μm particulate filtered from 330 ml of water from d =6.6 m. Five identical sets of raw data were averaged and processed with a variable smoothing grid: S c =15, S u,0 =10, S u,1 =15, λ H =0.1. The dotted contours denote FORC distributions that are significant at the 0.05 level. Full size image Coercivity distribution Magnetic coercivity distribution unmixing is another widely employed method for determining the amount of biogenic magnetic particles in natural sediments. Previously, magnetization curves measured from 26 sediment samples having different provenances have been decomposed into multiple coercivity distribution components. Two particular coercivity distribution components characterized by small dispersion parameters were hypothesized to represent magnetofossils [19] ( Fig. 6a ): the so-called BS-BM (median coercivity 43.3±1.1 mT, dispersion factor 0.191±0.023), and BH-BI (median coercivity 68.9±1.1 mT, dispersion factor 0.122±0.037). We measured detailed anhysteretic remanent magnetization (ARM) demagnetization curves on filters containing collections of uncultivated MTB from the Upper Pond water column and modelled their coercivity spectra (Methods). The coercivity distribution spectra of uncultivated MTB at different depths in the Upper Pond have remarkably similar shapes ( Fig. 6a ). The majority are characterized by left-skewed generalized Gaussian coercivity distributions with median 33.9±1.1 mT and dispersion factor 0.20±0.03 ( Supplementary Table 4 ). This result is significant for three reasons. First, prior associations of BS-BM and BH-BI with magnetofossils remains speculative because numerical inversion of magnetization curves through which they were originally conceived [19] and continuously presumed [16] , [48] , [49] , [50] , [51] has non-unique solutions. In addition, the coercivity distributions (characterized by skewness, median coercivity and dispersion factor) of diverse MTB types found in nature are poorly constrained. The similarity of the Upper Pond uncultivated MTB coercivity distributions to that of BS-BM strongly suggests the latter is closely related to magnetosomes. Second, the small dispersion parameters of both BS-BM and BH-BI are thought to reflect the tightly genetically controlled MTB biomineralization process in producing uniformly sized particles and therefore distinguishing them from non-biogenic magnetic particles [19] . Our results on collections of uncultivated MTB confirm this assertion, at least for the BS-BM component. Third, the skewed coercivity distributions that characterize uncultivated MTB point to the importance of modelling them as such, rather than symmetric distributions, so as to avoid the addition of coercivity distribution components that are not physically meaningful when quantifying the amount of magnetofossils. Both approaches are widely used [19] , [50] , [51] , [52] , [53] . Figure 6: Coercivity distribution and magnetosome size and shape. ( a ) Blue curves: ARM coercivity distribution of the water column samples from this study. Grey curves: hypothesized sedimentary magnetofossil coercivity distribution components BS-BM and BH-BI [19] . Black curves: averaged BS-BM and BH-BI. Thick light blue band: average coercivity determined from pulse-field experiments on individual greigite MTB from refs 57 , 59 . Thin magenta band: approximate median coercivity from a Miocene marl in ref. 38 containing greigite with similar crystal size distribution as MMP (‘many-celled magnetotactic prokaryote’), a greigite-producing MTB. Magenta curve: coercivity distribution determined from IRM acquisition curve unmixing from Pliocene sediment containing putative greigite magnetofossils [16] . ( b ) Aspect ratio (width/length) versus length for 377 magnetosomes imaged from 21 MTB in this study (blue dots). The grey dots ( n ~3000) are measured length and aspect ratio from putative magnetofossils extracted from marine and lacustrine sediments [55] . Blue and magenta boxes mark the length and aspect ratio ranges for MMP magnetosomes and greigite from the Miocene marl sample mentioned above, respectively, from ref. 38 . Magenta symbols denote magnetofossil shapes for the claimed oldest greigite magnetofossils from ref. 16 . Full size image The natural variability in FMR spectra displayed by uncultivated MTB explains why magnetofossil-bearing sediment samples, including the surface sediment from Upper Pond (containing ~77% magnetofossils, see Supplementary Fig. 10 ), do not always have spectral parameters that fall within the range defined by intact culture of magnetite-producing MTB characterized to date. Curiously, FMR spectra from several water column filter samples present double minima in the derivative spectra on the high-field side ( Fig. 4c ). This feature has been reported for titanomagnetite (TM10) [44] but never before observed in uncultivated MTB even though such a feature is intrinsic to chains of magnetosomes with mixed uniaxial and magnetocrystalline anisotropy [28] , [44] . An overall lack of low-field absorption peaks and uniformly high-field extended asymmetry ( A >1) characterize spectra from greigite-producing MTB in zone 3 ( Fig. 4c ). Such an asymmetry can be expected for systems dominated by a negative cubic magnetocrystalline anisotropy (<111> easy axis), which has been suggested as a probable case for greigite with aspect ratio >~0.75 (if elongated along <111>) [54] . In terms of magnetofossil detection, although the low-field absorption peaks remain a useful FMR trait in recognizing magnetite-producing MTB, our results from the water column, sediment trap and the surface sediment suggest that deviations of FMR empirical parameters from those of intact magnetite-producing MTB cultures characterized to date should not be inevitably taken to signify lower magnetofossil concentrations nor diagenetic alteration of MTB chains. The Upper Pond water column coercivity distribution findings presented in this study establish an unequivocal link between coercivity component BS-BM and MTB without complication from co-occurring magnetic mineral phases in typical sedimentary mixture or diagenetic alteration. The lack of the other supposed magnetofossil coercivity component, BH-BI, in the collection of uncultivated MTB from the Upper Pond can be understood by examining the particle size distribution determined from 377 magnetosomes imaged from 21 MTB cells (for example, Fig. 2f ) between d =5.0–6.2 m ( Fig. 6b ). The magnetosomes are within the single-magnetic domain size range [55] , [56] , their width and length distributions are roughly Gaussian in shape ( Supplementary Fig. 20a,b ), but their aspect ratios range from 0.4 to 1.0 and skewed towards equidimensional particles ( Supplementary Fig. 20c ). Putative magnetosomes with aspect ratio <0.4 have been reported in the literature [55] ( Fig. 6b ). There are also many known contemporary MTB strains that produce magnetite magnetosomes with aspect ratio <0.4, including all of the strains in the Nitrospirae phylum [35] . Moreover, coercivity component BH-BI have been detected in sediment samples containing putative elongated magnetite magnetosomes [50] , [51] . These magnetosomes have enhanced shape anisotropy and therefore a higher coercivity [57] , [58] . As such, we hypothesize that it is the absence of higher aspect ratio magnetosomes in Upper Pond that explains the absence of BH-BI. Coercivity distribution results from samples containing greigite magnetosomes in this study are in general agreement with pulse-field experiments on individual greigite MTB [57] , [59] and bulk coercivity of mixtures of greigite and magnetite MTB [7] ( Fig. 6a ). Although coercivity distributions were not determined from these previous studies, the range of coercivities measured to date from all known greigite MTB, 20–35 mT, is just slightly higher than the coercivity of ~13 mT [17] of contemporary sediment containing putative greigite magnetofossil. In contrast, these values are consistently much smaller than the ~78 mT median coercivity measured from Neogene sediments inferred to contain greigite magnetofossils [16] , [38] ( Fig. 6a ). As the range of aspect ratios of magnetic particles extracted from these Neogene sediments is similar to that of uncultivated magnetosomes from the Upper Pond ( Fig. 6b ), perhaps greigite magnetofossils are not the carrier of high-coercivity magnetic signals in these sediments. Instead, the narrow dispersion of this high-coercivity component, resembling that of BH-BI and attributed to controlled biomineralization [16] , could be the consequence of another natural process that also produce uniformly sized greigite particles: for example, authigenic greigite framboids (clusters) formation via sulphate reduction [60] . Another possibility is that an unidentified post-depositional chemical alteration mechanism could increase greigite magnetosome coercivity. In either case, enhanced interparticle interaction is involved. This is evident from the downward shifted central peak and the large FORC function width along the H u -axis measured from the Pliocene sediments claimed to host the oldest known greigite magnetofossils [16] . In contrast, the FORC diagram measured from MTB inhabiting d =6.6 m in the Upper Pond ( Fig. 5 and Supplementary Fig. 14 ) has a non-negligible contribution in the H u >0 range expected from the non-single chain arrangement of greigite magnetosomes ( Fig. 3b and Supplementary Fig. 1b ), but does not show a shift of the central peak. Similarly, no central peak shift was observed in a FORC diagram from contemporary sediments from the Baltic Sea containing putative greigite magnetofossils [17] . Our study points to confounding interpretations of BH-BI, either signifying greigite framboids, diagenetic alteration of greigite magnetosomes, or high aspect ratio magnetosome/magnetofossils. Through the use of an installed sediment trap, dead MTB exported out of the chemocline were collected over time. This, in conjunction with the water column ferrimagnetic particle concentration-dependent parameters shown in Fig. 2e and Supplementary Figs 12 and 18 allows us to determine an MTB population turnover rate of approximately once every 28.3 days (Methods). That is, neglecting seasonal variation, in 1 year, we can expect 12.9 times the MTB population living in the water column at the time of sampling to be exported out of d =7.0 m, the deepest depth where live MTB was observed by the hanging-drop assay and where the sediment trap was installed. This estimate is intrinsically inclusive of the MTB–protozoan interaction, as well as any dissolution that may or may not have occurred at d =3.9–7.0 m with or without assistance by the iron-chelating siderophores MTB produce. Given the MTB population turnover rate, the total amount of MTB Fe exported out of the chemocline is 15.3–18.2 μg Fe per cm 2 per year (Methods). This is a small fraction of the pyritic Fe flux (estimated 838 μg Fe per cm 2 per year) [40] in this particular euxinic basin with a high riverine Fe flux. However, the Fe flux in open euxinic basins, such as the Black Sea, is controlled mainly by turbidite frequency and the amount of remobilized shelf Fe [61] . As such, the flux of reduced Fe, estimated to be only 38±28 μg Fe per cm 2 per year [61] , is significantly smaller. Assuming a similar MTB population density, MTB-associated Fe flux could be a significant, and heretofore overlooked, component in the iron cycle in such open euxinic systems. Lastly, besides being an important component in the water column Fe cycle, MTB-associated Fe is also an important component of the sediment Fe cycle and sedimentary magnetic signal. From the MTB population turnover rate and the ARM profile from the water column, the contribution from MTB to the surface sediment magnetic signal in 1 year, assuming none of the exported magnetosomes are altered by diagenesis, is 8.15 × 10 −4 Am 2 m −2 per year (Methods). A simple comparison between this expected signal and the fraction of surface sediment ARM carried by magnetosomes deduced from coercivity component analysis, accounting for accumulation rate, 3.45 × 10 −4 Am 2 m −2 per year, show that up to 42% of magnetosomes exported out of the chemocline remain in the surface sediment after 12.5 years of exposure to sulphidic water (Methods). Further, if all zone 1 and 50% of zone 2 magnetosomes are magnetite in composition, and all zone 3 and the other 50% of zone 2 magnetosomes are greigite in composition, then of the 42% of magnetosomes that are preserved, 44–94% can be magnetite and 6–56% can be greigite (Methods). Our analysis demonstrates that magnetosomes can be preserved in euxinic basin sediments that had been immersed in sulphidic water for a short term, which is a prerequisite if they are to be used as biomarkers of ancient euxinia. Further studies are required to understand the longer-term preservation potential and diagenetic alteration pathway, although a previous study on the nearby Lower Pond sediment does show substantially retained bulk ARM, carrier unknown, dating as far back as 1600 A.D. [62] . Employing similar approaches to the one we have presented in this study to investigate other stratified euxinic and ferruginous systems will allow for more robust interpretation of sedimentary magnetic signal that reflect the property of diverse and naturally occurring MTB, and can lead to better understanding of their contribution to the biogeochemical cycling of iron and other important elements. Water column profile and sample collection From an anchored boat, DO and Eh were monitored on 15 September 2012 by a calibrated YSI556 electrode. Winkler titration independently confirmed negligible DO from several discrete water depths with DO below YSI556 detection limit. For the water collection, the intake of a Geotech pump was taped to a L-shaped aluminum bracket covered by electrical tape, which was fixed to the YSI556 electrode. Water from each sampling depth was collected into one 2-l plastic bottle and one 250-ml bottle filled to their maximum capacity at the rate of ~3 min l −1 . The bottles were kept in coolers with ice during the ~2 h transit between the sampling site and the lab. A simple sediment trap was installed in the Upper Pond water column for ~10 days (14–24 September 2012; Supplementary Fig. 2 ). In each of the two plastic trap cylinders, inner diameter 2.75′′ (6.985 cm), the estuary surface water was used to fill the cylinders up to a pre-marked level, such that when 1 litre of saturated NaCl solution (to provide density contrast) with 1 g HgCl 2 (to retard cell degradation) was placed in the cylinder from the bottom using a clear vinyl tubing with a plastic funnel attached, the cylinders were filled to the top. The sediment trap was suspended at d =7.0 m (the deepest depth at which a preliminary survey on 3 September 2012 showed the presence of MTB and magnetically responsive protists). The sediment trap was held upright by one subsurface buoy and one surface buoy and moored. Surface sediment samples were obtained by an Ekman dredge lowered from an anchored boat. Retrieved sediment was frozen within 2 h of collection, freeze-dried and placed in a tightly sealed container until measurement. Live cell hanging-drop assay For the observation of MTB morphotypes, hanging-drop assay, as described in ref. 35 and illustrated in Supplementary Fig. 3 , was performed on water sample collected in the 2-l bottles at every depth. One representative 20 μl droplet was taken from gently shaken bottles. The south pole of a bar magnet was placed at one side of the droplet on a Zeiss Scope A1 compound microscope stage. Images were taken with a digital camera attached to the microscope at × 100 magnification. Filtration and sample sets After hanging drop assay, three sets of samples were prepared by ‘dead end’ vacuum filtration ( Supplementary Fig. 4a ). One set of samples intended for remanent magnetization measurements was prepared from filtering 1 litre of water from each depth sequentially through four 47-mm diameter filters with pore size 0.8–8 μm (glass fiber pre-filter), 1.2, 0.45 and 0.22 μm. A second set of samples intended for hysteresis and FMR measurements was prepared by filtering 250 ml of water from each depth through one 47-mm diameter filter with pore size 0.22 μm. The third set of sample intended for FORC measurements was prepared by filtering 440 ml of water taken from d =6.6 m through one 47-mm filter with pore size 0.22 μm. To minimize oxidation, all filters were frozen immediately, freeze-dried within a day and sealed with a store-bought vacuum food saver along with desiccant until measurements and between measurements. On retrieval of the sediment trap, the bottom-most 1 litre in the sediment trap was removed from a bottom valve on the sediment trap cylinders. The rest of the water in the cylinder appeared clear with little suspended material compared with the collected fraction. The collected water was transported on ice (~2-h transit time) and centrifuged at 4 °C for 45 min at 8,500 r.p.m. Approximately 99% of supernatant was filtered first through a glass fibre pre-filter (47 mm diameter, pore size 0.8–8 μm), while ~10 ml of the supernatant and deionized water was used to re-suspend the precipitate (‘pellet’), which were then also filtered through the glass fibre pre-filter. All filtrate from the glass fibre pre-filter was then passed through three 47 mm filters with pore size 1.2, 0.45 and 0.22 μm. Again, to minimize oxidation, all filters were frozen immediately and freeze-dried within a day, sealed with a store-bought vacuum food saver along with desiccants until and between measurements. Remanent magnetization and coercivity distribution From the first sample set, four filters from each water column depth and four filters from the sediment trap were folded and tightly placed in plastic paleomagnetic cubes. To evaluate the background signal, a ‘blank sample’ was constructed from four un-used filters, pore size 0.8–8, 1.2, 0.45 and 0.22 μm. ARM and isothermal remanent magnetization (IRM) were measured with a SQUID rock magnetometer (2G Corp. SRM) fitted with an inline alternating-field degausser and DC magnetizer in the Massachusetts Institute of Technology, Paleomagnetic Laboratory. ARM was acquired with AF max =200 mT, DC=0.1 mT, while IRM was imparted with DC=200 mT, both along a single axis. AF demagnetization of ARM (along the same single axis) was measured at 98-log-spaced steps between 0 and 200 mT by an automated measurement sequence, that is, elapsed time between demagnetization steps stayed constant for all samples. ARM susceptibility ( χ ARM ) was calculated from the intensity of ARM normalized by the DC biasing field. The sample-to-blank ratios (S/B) for ARM (AF=0) and IRM are shown in Supplementary Fig. 5 . The signal from the blank sample was subtracted from the bulk ARM and IRM data before they are presented as filtered-water-volume-normalized magnetic moment ( Fig. 2e ) and χ ARM /IRM ratio ( Supplementary Fig. 6 ). The coercivity distribution was calculated from ARM AF demagnetization curves using CODICA and modelled using a flexible generalized skewed Gaussian function by GECA (ref. 53 and Supplementary Methods ). Hysteresis and FORC Filters from the second (all depths) and third ( d =6.6 m) sample sets were folded in half, with the two halves glued together by a small amount of Elmer’s glue. A ceramic knife was used to cut half (containing >0.22 μm particulate fraction from 125 ml for each water depth) or 3/4 (containing >0.22 μm particulate fraction from 330 ml for d =6.6 m) of the filter into 4.5- to 5.5-mm squares, which were then stacked and glued together and allowed to dry in air completely ( Supplementary Fig. 4b ). A blank sample was constructed the same way with a new 0.22-μm filter. For the sediment trap sample, the four filters in the paleomagnetic cube for remanent magnetization were unfolded and 1/8 of each filter (or the equivalent of particulate accumulated over 1.25 days) were also cut into 4.5-mm squares and glued together. Hysteresis loops (three to six replicates) for the water column (second set) and sediment trap filters were made with an alternating gradient force magnetometer (AGFM) at Princeton Measurement Corp., Princeton, New Jersey. Specimen anisotropy was checked by hysteresis loop measurements made on ‘filter stacks’ with the filter paper plane oriented parallel and perpendicular to the applied field. The similarity between the hysteresis loops measured from these two orientations indicates very small specimen anisotropy as expected from the ‘dead end’ filtration method ( Supplementary Figs 4a and 11 ). Five sets of FORC from d =6.6 m were collected from the third filter sample set and measured with an AGFM at the Institute for Rock Magnetism, University of Minnesota. Both AGFM and VSM were calibrated by a standard daily. For AGFM measurements, each sample was auto-tuned in a 500-mT applied field. For better temporal stability, a mechanical gain of 2 was specified and the higher of the two operating frequency choices offered by the instrument control software (MicroMag) was used. Hysteresis and FORC parameters used to collect the data are listed in Supplementary Table 3 . The measured hysteresis loops and estimates of saturation magnetization ( M s) for all samples were obtained after correction for the diamagnetic slope at high field as described in ref. 63 . Supplementary Table 4 summarizes M s and signal-to-noise (s/n) ratio for the ferromagnetic hysteresis component averaged from repeated measurements. The hysteresis loop measured from an un-used 0.22-μm filter has unreasonable negative M s after correction due to its weak signal; hence, no blank subtraction was performed on filter samples. M s as a function of water depth is shown in Supplementary Fig. 12 . Five sets of FORC acquired with identical experimental parameters on the filter sample from d =6.6 m were averaged and processed by FORCinel version 2.01 (ref. 64 ) by both equally spaced smoothing grid and a variable smoothing grid described in ref. 26 . For the latter, the software offers the possibility to add statistical significance threshold contours described in ref. 65 . For the former, the choice of the tricube weighted loess smoothing factor (SF) was determined by inspecting the SF versus s.d. of the residual and SF versus first derivative of s.d. of the residual between the (averaged) measured data and the smoothed FORC data ( Supplementary Fig. 13 ). SF=15 was the optimum value determined by the software from such residual analyses (for SF=3–15 in step of 1), and the corresponding FORC diagram is shown in Supplementary Fig. 14 . For the variable smoothing grid, we used S c =15, S b,0 =10, S b,1 =15, λ H =0.1 (see ref. 26 for parameter definitions). Ferromagnetic resonance From the second sample set, the same stack of 5-mm square samples from a few depths used for hysteresis measurements were re-used for FMR, while 4.5 mm squares were cut from the other half of the 47 mm filters from the second sample set for others. For the sediment trap measurements, the sample for hysteresis measurement was cut in half (~1/16 of original specimen, equivalent to particulate accumulated over 0.625 days). Surface sediment (0.1303, g) was used for the FMR measurement. The FMR measurements were made at X-band with a Bruker EPR Spectrometer (Elexsys E580) in the Department of Chemistry, Rutgers, The State University of New Jersey. Except for the surface sediment sample that was measured in a dedicated EPR tube (Wilmad 710-SQ-250M), the stacked filters shared an EPR tube (Wilmad 748-PQ-7) and were swapped in and out of the tube between measurements throughout the experiment. Microwave absorption was measured as a function of applied field. Two to four scans were performed per sample (parameters are summarized in Supplementary Table 5 ), with periodic re-measurement of empty EPR tube to check for possible contamination [65] . The blank sample, constructed from an un-used 0.22 μm filter and Elmer’s glue in the same manner as for the water column and sediment trap samples contain trace amounts of ferromagnetic material, attested by its similar total FMR absorption as an empty EPR tube ( Supplementary Fig. 15a ). Repeated measurements of empty EPR tube throughout the experiment suggest that contamination of the tube is negligible ( Supplementary Fig. 15a,b ). The FMR absorption spectra were processed as follows (in order): (1) the blank signal was subtracted from the raw data, (2) drift was corrected ( Supplementary Fig. 16 and 17a ) and (3) high-frequency paramagnetic peaks were removed by Fast Fourier Transform (FFT) smoothing ( Supplementary Fig. 17a ). The blank signal subtraction was performed in order, that is, samples measured after t =0 and before t =1 were subtracted by blank measured at t =0, which denotes the start of the experiment. The drift correction was performed by subtracting the FMR absorption by a baseline fitted with data from 10.6 to 11.1 mT and 608.8 to 609.4 mT. The FFT smoothing was performed by removing data with frequencies above 0.01 to 0.96 times the mean frequency of the discrete Fourier-transformed FMR absorption data. Examples are given in Supplementary Fig. 17b,c . Total FMR absorption obtained from processed spectra as a function of water depth is presented in Supplementary Fig. 18 . Empirical parameters used to characterize FMR spectra were calculated from the final FFT smoothed field versus absorption data following the approach in refs 20 , 21 , 22 and graphically illustrated in Supplementary Fig. 19 . The results are summarized in Supplementary Table 6 for all samples, except for the water column samples from d <3.9 m having a low sample-to-blank total absorption ratio of ~1 ( Supplementary Fig. 16c ). Analytical microscopy TEM samples were prepared from enriched North-seeking MTB. The cells were fixed overnight with electron microscopy-grade glutaraldehyde (final fixative concentration 2.5%). We washed the sample several times with phosphate buffer adjusted to neutral pH (0.1 M). To prepare the TEM grid, the sample was deposited on a polyvinyl butyral-coated Cu 200 mesh grid inside a humid chamber. The grids were allowed to dry in air completely and stored in desiccator until and in between observations. Images for particle size analysis was taken with a Philips CM10 TEM equipped with a digital camera (Olympus SIS MegaView G2) in the Microscopy Unit, Macquarie University. Images of two-dimensional particle projections were fitted with ellipses, following the method in refs 38 , 66 . The major and minor axes are reported as length and width and presented in Fig. 6b , and the width, length and aspect ratio histograms are presented in Supplementary Fig. 20a–c , respectively. Error from such analyses arise from the unknown orientation of particles with respect to the TEM grid and from the ellipse approximation; both are apparently small [38] , [66] . Chemical composition of magnetosomes in two MTB from d =5.8 m and d =6.2 m were determined with a JEOL 2010F TEM in the Nuclear Materials Modeling and Characterization Programme, Australian Nuclear Science and Technology Organisation. All EDS spectra were collected with a live time of 30 s. Owing to the close proximity of magnetosome particles with one another and their position within the intact bacterial cell, the X-ray point analyses on individual particles probably contain signals from neighbouring particles and the cell membrane. MTB population turnover and Fe flux MTB population turnover rate (that is, the amount of time for all MTB present in the water column at any instantaneous time to die and fall out of the chemocline) was calculated from ferromagnetic particle concentration-dependent IRM, ARM, FMR total absorption and M s from the depth integrated water column filter measurements and the sediment trap measurements. The depth integrated signal was calculated for d =3.9–7.0 m only, where live MTB were observed during hanging-drop assay ( Fig. 2b ). An example of the MTB turnover rate calculated from the IRM signal is given in the Supplementary Methods . The results are summarized in Supplementary Table 7 . We calculate the flux of MTB Fe (that is, the amount of MTB iron that is exported out of the chemocline per year) with the following parameters: Depth-integrated M s ( d =3.9–7.0 m; from Supplementary Table 7 )=0.0015 Am 2 m −2 . Average MTB turnover rate ( Supplementary Table 7 )=every 28.3 days or 12.9 times per year. M s of magnetite (ref. 67 )=90 Am 2 kg −1 . M s of greigite (ref. 68 )=59 Am 2 kg −1 . As Pettaquamscutt River Estuary is stratified year-round (complete water column overturn is not considered here), neglecting seasonally variations, the total MTB Fe flux out of the chemocline is 15.3 (as magnetite) −18.2 (as greigite) μg Fe per cm 2 per year. Magnetosome preservation We compare the flux of magnetosomes (ARM, Am 2 per cm 2 per year) exported out of the chemocline with the surface sediment magnetic signal to estimate the preservation of magnetosomes. Without any diagenesis either in the sulphidic water column or in the surface sediment exposed to sulphidic water, using the averaged MTB turnover rate from Supplementary Table 7 (every 28.3 days or 12.9 times per year) and the d =3.9–7.0 m depth integrated ARM signal (6.3289 × 10 −5 Am 2 m −2 ), we can expect magnetosomes to contribute 8.15 × 10 −4 Am 2 m −2 per year to the surface sediment ARM signal. The retrieved surface sediment sample represents sediment mixture from the top ~5 cm of the sediment. Using the following parameters we can calculate the magnetosome flux (ARM Am 2 cm −2 per year) in the surface sediment: Sedimentation rate (averaged from 1962–2005 in ref. 69 ): 0.004 m per year. Dry sediment density (averaged from the top 6.25 cm of a sediment core in ref. 69 ): 2.12 × 10 3 kg m −3 . Porosity (averaged from the top 6.25 cm of a sediment core in ref. 69 ): 0.9529. Accumulation rate=(dry sediment density) × (sedimentation rate) × (1-porosity): 0.399 kg m −2 per year. ARM from magnetosomes in the surface sediment (77% of 1.1 × 10 −3 Am 2 kg −1 estimated from ARM coercivity unmixing, Supplementary Fig. 10 ): 8.5 × 10 −4 Am 2 kg −1 . Therefore, the actual magnetosome flux to the surface sediment is 3.45 × 10 −4 Am 2 m −2 per year, or a 42% preservation. Some fraction of the 58% of magnetosomes that are not preserved in the surface sediment can be attributed to reductive dissolution of magnetite magnetosomes in sulphidic water, which we estimate using the magnetite dissolution rate law from ref. 12 : where t is time in years, C mag is the concentration of magnetite, k is the reaction rate constant, C s is the sulphide concentration, A mag is the specific surface area of magnetite grain and the following parameters: Maximum amount of time the surface sediment we recovered has been exposed to sulphidic water: (sedimentation rate) × (5 cm)=12.5 years. C s of Upper Pond, Pettaquamscutt River Estuary (ref. 40 ): 4 mM. k : −1.5 × 10 −6 (ref. 70 ) to −1.1 × 10 −5 (ref. 12 ). A mag : calculated using the Knud Thomsen’s formula for surface area of prolate spheroid from magnetosome particle size measured from d =5.0–5.4 m in the water column (semi-axis 25.8±8.6 and 23.1±11.5 nm), volume for prolate spheroid and magnetite density of 5.175 g cm −3 , A mag =3.27 × 10 4 cm 2 g −1 . According to the above, C mag_final = e −bt , where b =0.0981–0.7194 depending on k , and over 12.5 years, on average 11.2–57.7% of magnetite magnetosomes that settled through the sulphidic water column and immersed in sulphidic water in the surface sediment are expected to dissolve. The amount of magnetite versus greigite magnetosome flux exported out of the chemocline was estimated by assuming that all ARM signal between d =3.9–5.0 m are from magnetite magnetosomes, ARM signal between d =5.0–6.0 m are from magnetite magnetosomes (50%) and greigite magnetosomes (50%), and all ARM signal between d =6.0–7.0 m are from greigite magnetosomes. The depth integrated ARM for magnetite and greigite magnetosome flux breakdown are summarized in Supplementary Table 8 . Compared with the actual magnetosome flux to the surface sediment (3.45 × 10 −4 Am 2 m −2 per year ), we estimate between 4.8% (if 1.540 × 10 −4 Am 2 m −2 per year magnetite magnetosome survived dissolution) to 42% (if 3.232 × 10 −4 Am 2 m −2 per year magnetite magnetosome survived dissolution) of the greigite magnetosome flux out of chemocline is preserved in the surface sediment after 12.5 years. How to cite this article: Chen, A. P. et al. Magnetic properties of uncultivated magnetotactic bacteria and their contribution to a stratified estuary iron cycle. Nat. Commun. 5:4797 doi: 10.1038/ncomms5797 (2014).